Genetic requirements for repair of lesions caused by single genomic ribonucleotides in S phase 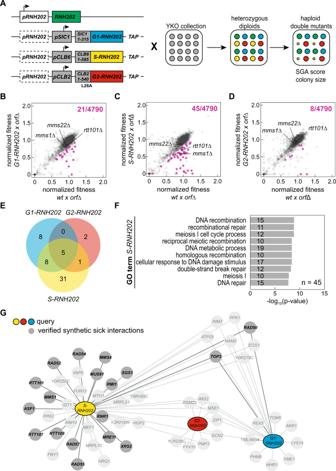Fig. 1: SGA screen identifies network of genes required for rNMP-derived lesion tolerance in S phase. AFor the SGA analysis, the illustrated three query strains (G1-RNH202,S-RNH202,and G2-RNH202) were crossed to the non-essential yeast knockout (YKO) collection. The heterozygous diploids were sporulated and fitness of the resulting haploid double mutants was scored based on their colony size. The outcome was compared to the corresponding scores from the wild type (RNH202) cross. For each genotype, four replicates per strain were generated and analyzed. Scheme was created using Adobe Illustrator.B–DScatter plots of normalized double mutant fitness for the queries compared to wild type (wt). The three queries with cell cycleRNH202alleles compared to the wild type control (wt). Each data point represents a single mutant in the YKO collection. Significant synthetic sick interactions (fitness query xorfΔ wt xorfΔ <0.8,p< 0.05 in a t-test, corrected for multiple testing using the Benjamini-Hochberg method) are highlighted in magenta. Crosses withmms1Δ,mms22Δ andrtt101Δ mutants are indicated. Top right, total number of significant synthetic sick interactions.EVenn diagram of the number of synthetic sick interactions for the three queries with the cell cycle restrictedRNH202alleles.FGO term enrichment analysis for synthetic sick interactions of theS-RNH202query. Only Biological Process GO terms are shown, top 10 terms byp-value in a hypergeometric test.GNetwork summary of the synthetic sick interactions for the three queries with the cell cycleRNH202alleles. Genes mapped to the GO term „DNA metabolic process” are highlighted in grey. We could exclude genes with linkage to thernh202Δ locus, and manual tetrad dissection identified false positives (Supplementary Data1). These false positive hits were excluded from the network (faint appearance in the scheme). Single ribonucleoside monophosphates (rNMPs) are transiently present in eukaryotic genomes. The RNase H2-dependent ribonucleotide excision repair (RER) pathway ensures error-free rNMP removal. In some pathological conditions, rNMP removal is impaired. If these rNMPs hydrolyze during, or prior to, S phase, toxic single-ended double-strand breaks (seDSBs) can occur upon an encounter with replication forks. How such rNMP-derived seDSB lesions are repaired is unclear. We expressed a cell cycle phase restricted allele of RNase H2 to nick at rNMPs in S phase and study their repair. Although Top1 is dispensable, the RAD52 epistasis group and Rtt101 Mms1-Mms22 dependent ubiquitylation of histone H3 become essential for rNMP-derived lesion tolerance. Consistently, loss of Rtt101 Mms1-Mms22 combined with RNase H2 dysfunction leads to compromised cellular fitness. We refer to this repair pathway as n ick l esion r epair (NLR). The NLR genetic network may have important implications in the context of human pathologies. Single ribonucleoside monophosphates (rNMPs) are present in the genomic DNA (gDNA) of yeast and human cells. The budding yeast Saccharomyces cerevisiae incorporates about 10,000 rNMPs into the genome per cell cycle [1] . DNA polymerases incorporate rNMPs during the DNA replication process. The double-stranded context of gDNA does not permit the reduction of the 2′-hydroxyl (2′-OH) group of the misincorporated rNMP, hence its presence can lead to single-strand DNA (ssDNA) breaks (nicks) of the sugar-phosphate backbone that result in replication fork collapse and the formation of single-ended double-strand breaks (seDSBs) in S phase. In addition, genomic rNMPs themselves hinder the passage of DNA polymerases and cause replication stress; a phenotype conserved from yeast to human cells [1] , [2] , [3] , [4] , [5] , [6] . Therefore, it is critical to remove rNMPs in a timely manner to prevent rNMP-derived genomic instability. RNase H2 is the central ribonucleotide excision repair (RER) enzyme in yeast and mammalian cells [7] . The majority of rNMPs that have been incorporated into nascent gDNA during DNA replication in S phase can be removed in the subsequent G2 phase [8] . When RER fails, topoisomerase 1 (Top1) can process genomic rNMPs. Top1 action at rNMPs is however associated with genomic instability due to error-prone branching in the Top1 pathway [9] , [10] . Even in the presence of RER, Top1 nicks some rNMPs [11] , but the precise interplay between RNase H2 and Top1 remains to be elucidated. Nonetheless, timely elimination of genomic rNMPs is crucial, and defective RER is associated with human diseases such as chronic lymphocytic leukemia and prostate cancer [6] . RNase H2 is a trimeric enzyme in yeast ( RNH201, RNH202, RNH203 ) and mammalian cells (RNASEH2A, RNASEH2B, RNASEH2C) [7] . We previously engineered cell cycle regulated alleles for the RNH202 gene to restrict expression of the enzyme to either the S or G2 phase of the cell cycle [8] . In addition to the finding that expression of RNH202 exclusively in G2 was sufficient to suppress RER defects, we observed an unexpected fitness defect when RNase H2 activity was restricted to S phase [8] . Yeast with S phase expressed RNH202 ( S-RNH202-TAP, referred to as S-RNH202 ) experienced toxicity caused by nicking of the gDNA and relied on the homology-directed repair (HDR) factor Rad52 for survival [8] . The decreased fitness of the S-RNH202 strain was strongly exacerbated in presence of the pol2-M644G allele, a Polymerase ε (Pol ε) mutant that incorporates 10-fold more rNMPs [1] , [12] . Notably, the S-RNH202 phenotype was independent of Top1 activity suggesting that the RNase H2-mediated nicking of rNMPs in the S phase can cause toxic seDSBs during replication. Surprisingly, rNMP accumulation can be tolerated in the absence of both RER and Top1 pathways. This is evidenced by the viability of budding yeast lacking Top1 and expressing an allele of RNase H2 that is deficient in RER (but proficient in R-loop removal) [13] . This implies that cells can either tolerate the presence of replication stress and DNA damage from rNMPs, or that there might be other rNMP lesion repair pathways that act independently of RNase H2 and Top1 (discussed in ref. [14] ). In this study, we set out to get a better understanding of how rNMP-induced DNA lesions are repaired, when the nicking occurs during, or prior to, DNA replication. We used the S-RNH202 allele as a molecular tool to promote nicking of genomic rNMPs in S phase [8] . Using synthetic genetic array (SGA) technology [15] , we demonstrate that the RAD52 HDR epistasis group, the histone remodelers Asf1 and Rtt109, the STR (Sgs1-Top3-Rmi) complex, the Mus81-Mms4 resolvase, and the E3-Ubiquitin ligase complex Rtt101, Mms1, and MmsS22 are all required for the tolerance of rNMP-derived nicks during S phase. These factors comprise a Top1-independent, rNMP-derived n ick l esion r epair (NLR) pathway. We also found that histone H3 ubiquitylation by the replisome-associated Rtt101 Mms1-Mms22 complex is critical for NLR in high rNMP conditions, pointing to a role for chromatin remodelling in NLR. We summarize our genetic data in a model that likely represents the molecular processes in the NLR repair pathway. When a replication fork runs into an rNMP-derived strand nick, whether it be on the leading or lagging strand, a seDSB is formed. Rtt101-dependent post-translational modifications at chromatin and perhaps elsewhere then promote HDR. The STR and Mus81-Mms4 complexes are needed to provide resolution of the recombination intermediates. Importantly, we also report a negative genetic interaction between RTT101 and the complete loss of RNase H2, which becomes synthetic lethal when the genomic rNMP load increases. These data in yeast may provide therapeutic insights and alternatives for human cancer treatment in genetic contexts where RNase H2 is dysfunctional such as RER-deficient cancers [6] . Genetic screen identifies a network required for rNMP-derived lesion tolerance in S phase We employ the S-RNH202-TAP allele (from here on referred as S-RNH202 ) as a tool to endogenously nick genomic rNMPs in S phase. Restricting the expression of RNase H2 to S phase also results in the accumulation of genomic rNMPs, which supports the notion that the bulk of RER occurs outside of the S phase. Indeed, the rNMP load is similar in S-RNH202 as it is in RER-deficient strains [8] . Consistently, the S-RNH202 allele has a similar rate of mutagenesis as the RNase H2 deletion ( rnh202 Δ) in the presence of the pol2-M644G allele, a Polymerase ε (Pol ε) mutant that increases the rNMP load by 10-fold [12] (Supplementary Fig. 1A ). RNase H2 deletion and S-RNH202 expressing strains share not only the same amount of genomic rNMPs, and the same mutagenesis rate but also are both highly sensitive towards hydroxyurea (HU) (in the pol2-M644G background) (Supplementary Fig. 1B ). Methyl methane sulfonate (MMS) stabilizes R-loops which are potentially toxic RNA-DNA hybrids that are removed by RNase H1 and RNase H2 [8] . In the presence of MMS, the rnh1 Δ rnh201 Δ double mutant and rnh1 Δ S-RNH202 double mutant are inviable (Supplementary Fig. 1C ). Therefore, both canonical RNase H2 functions, R-loop removal and RER, likely occur outside of S phase. Taken together, these data suggest that employing the S-RNH202 allele as an enzymatic tool to endogenously nick genomic rNMPs recapitulates many phenotypes of an RNase H2 deletion, and suggests that many problems associated with loss of RER are due to rNMP nicking during DNA replication. Therefore, the S-RNH202 allele is relevant both in terms of understanding rNMP repair during RER deficiency (rNMP hydrolysis in S phase) and in canonical RER, when RNase H2 nicked rNMPs are not repaired in a timely manner and are encountered in the following S phase. To identify factors involved in repair of rNMP-derived lesions occurring in S phase we performed a synthetic genetic array (SGA) analysis with cell cycle restricted alleles of RNH202 in the budding yeast Saccharomyces cerevisiae (Fig. 1A ). We generated G1-, S-, and G2-restricted alleles of RNH202 in the query background (Supplementary Fig. 1D, E ). Then, we crossed the three queries along with the wild type control to the haploid yeast knockout collection (YKO) of non-essential genes. We derived haploid double mutants and determined their fitness by measuring colony size (Fig. 1A ). We compared the hits of each RNH202 cell cycle allele with the wild type RNH202 control to identify allele-specific genetic interactions (representative examples Supplementary Fig. 1F– H ). Out of 4790 gene knockouts included in the screen, we identified 21 synthetic sick interactions for the G1-RNH202 allele (Fig. 1B ), 45 for the S-RNH202 allele (Fig. 1C ), and eight for the G2-RNH202 allele (Fig. 1D ). Of those hits, five genes were essential to support normal colony size among all three alleles (Fig. 1E ). Gene Ontology (GO) revealed that the GO processes related to “DNA recombination” and “DNA repair” were enriched among the 45 synthetic sick interactions of the S-RNH202 allele (Fig. 1F ). This is in line with our previous finding that the HDR factor Rad52 is essential in the S-RNH202 genetic background [8] . We tested all candidates by manual tetrad dissection and curated the genetic interaction network accordingly (Supplementary Data 1 , Supplementary Fig. 1I, J , and Fig. 1G ). Among the synthetic sick interactions unique to the S-RNH202 allele, we identified RAD52 epistasis group genes ( RAD52, RAD54, RAD55, RAD57 ) consistent with our previous report [8] , the MUS81-MMS4 nuclease complex, the SGS1-TOP3 - RMI1 (STR) helicase complex, the MRE11-XRS2-RAD50 (MRX) nuclease complex, the nucleosome assembly factors RTT109 and ASF1 and the RTT101 MMS1 ubiquitin ligase (Supplementary Fig. 1I and Fig. 1G ). None of the G2-specific synthetic sick interactions was confirmed by manual tetrad dissection and thus were false-positives, consistent with canonical RER occurring in this phase of the cell cycle (Supplementary Fig. 1J ). Interestingly, translesion synthesis appears to not play a role for maintaining S-RNH202 fitness (Supplementary Fig. 1K ). Fig. 1: SGA screen identifies network of genes required for rNMP-derived lesion tolerance in S phase. A For the SGA analysis, the illustrated three query strains ( G1-RNH202 , S-RNH202 , and G2-RNH202 ) were crossed to the non-essential yeast knockout (YKO) collection. The heterozygous diploids were sporulated and fitness of the resulting haploid double mutants was scored based on their colony size. The outcome was compared to the corresponding scores from the wild type ( RNH202 ) cross. For each genotype, four replicates per strain were generated and analyzed. Scheme was created using Adobe Illustrator. B – D Scatter plots of normalized double mutant fitness for the queries compared to wild type (wt). The three queries with cell cycle RNH202 alleles compared to the wild type control (wt). Each data point represents a single mutant in the YKO collection. Significant synthetic sick interactions (fitness query x orf Δ wt x orf Δ <0.8, p < 0.05 in a t-test, corrected for multiple testing using the Benjamini-Hochberg method) are highlighted in magenta. Crosses with mms1 Δ, mms22 Δ and rtt101 Δ mutants are indicated. Top right, total number of significant synthetic sick interactions. E Venn diagram of the number of synthetic sick interactions for the three queries with the cell cycle restricted RNH202 alleles. F GO term enrichment analysis for synthetic sick interactions of the S-RNH202 query. Only Biological Process GO terms are shown, top 10 terms by p -value in a hypergeometric test. G Network summary of the synthetic sick interactions for the three queries with the cell cycle RNH202 alleles. Genes mapped to the GO term „DNA metabolic process” are highlighted in grey. We could exclude genes with linkage to the rnh202 Δ locus, and manual tetrad dissection identified false positives (Supplementary Data 1 ). These false positive hits were excluded from the network (faint appearance in the scheme). Full size image Surprisingly, only two hits were confirmed with the G1-RNH202 allele, both involved in the HDR pathway. The G1 allele is the least tightly regulated of all RNH202 alleles (Supplementary Fig. 1E ). To exclude that the complementation of G1-RNH202 was due to a weak expression of the G1 allele into S phase we performed synchronization experiments combined with induced-expression of RNase H2 only in G1 phase. These unpublished data support the spotting in Supplementary Fig. 1B and will be part of the future characterizing of RNase H2 activity in the G1 phase. In summary, the results with the G1-RNH202 allele indicate that RNase H2 initiated rNMP-repair may also take place in G1 phase. However, we could envisage that HDR is needed to an extent, in the case that nicked rNMPs from G1 are passed into the following S phase where these nicks again meet the replisome and ultimately would form seDSBs. A recent study identified genetic interactions when RNase H2 is absent, and included both non-essential gene deletions as well as essential mutants from the temperature-sensitive yeast collection [16] . 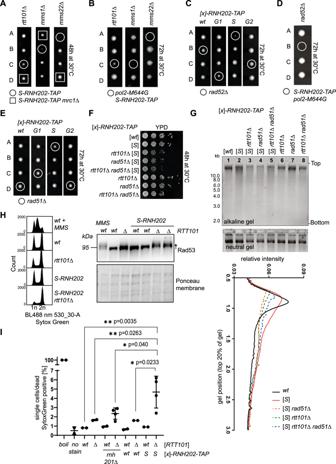Fig. 2: Rtt101, histone modifiers and HDR factors promote cell viability when genomic rNMPs are hydrolyzed in S phase. ATetrads from Rtt101Mms1-Mms22complex-deficient diploid strains in combination withS-RNH202-TAPrevealed smaller colony sizes (colonies in circles). The genetic suppressor ofrtt101Δ,mrc1Δ is sufficient to fully reverse the growth phenotype19(colonies in squares).BTetrads from dissections of Rtt101Mms1-Mms22complex-deficient diploid strains in theS-RNH202-TAP pol2-M644Ggenetic background augmented the sickness. Thertt101ΔS-RNH202-TAP pol2-M644Glethality was less penetrant compared to themms1Δ andmms22Δ mutants, but after propagating, these small colonies were mostly inviable or acquired suppressor mutations.CTetrad dissections ofrad52Δ withRNH202-TAPcell cycle alleles demonstrates that theS-RNH202-TAP rad52Δ double mutant is inviable.DThe phenotype from (C) was exacerbated when increasing the rNMP load (pol2-M644G).EThe tetrads forRAD51deletion with all cell cycle alleles ofRNH202shows that theS-RNH202 rad51Δ double mutant is sick but viable.FSpot assay shows epistasis betweenS-RNH202-TAP rtt101Δ andS-RNH202-TAP rad51Δ double mutants and theS-RNH202-TAP rtt101Δrad51Δ triple mutant.GAlkaline gel electrophoresis of the genotypes used in F) showed epistasis in terms of gDNA fragmentation betweenS-RNH202-TAP rtt101Δ andS-RNH202-TAP rad51Δ double mutant and theS-RNH202-TAP rtt101Δrad51Δ triple mutant (compare lanes 3, 4, 5). The neutral gel serves as control for gDNA purity and integrity. Two alkaline gels revealed the same result.HWestern blot analysis of checkpoint status by phospho-shift analysis of Rad53. The DNA profiles showed a 2n peak accumulation in line with the activated Rad53 checkpoint.IViability analysis of exponential cultures stained with SYTOX Green shown as Scatter dot blot (line = mean, error bars = SD). “Boil” is the boiled positive control representing 100% dead hence SYTOX green positive cells. The unstained wild type sample serves as background control. Statistical analysis with GraphPadPrism8 (multiple comparison ANOVA test),n= 2 for all samples exceptrnh201Δrtt101Δ andS-RNH202-TAP rtt101Δ n = 4 samples. Source data are provided as a Source Data file. We identified seven genetic interactions that are shared between RER-deficiency ( rnh201 Δ) and S phase restricted RNase H2 ( S-RNH202 ) (Supplementary Fig. 2A, B ). Plotting the genetic interaction String network of the complete hit list from the Chang et al. study allowed us to identify a gene cluster comprising eleven genes, including the MRX complex ( MRX - RAD50 - XRS2 )(Supplementary Fig. 2C, D , red circle ). Of those eleven genes of the “MRX cluster”, seven genes constitute the identified non-essential shared hits (Supplementary Fig. 2A, B ). We could validate the other four genes in the MRX cluster as true synthetic sick interactions with S-RNH202 (Supplementary Fig. 2E ). In conclusion, RER-deficiency and S-RNH202 require the same genetic network to maintain fitness, i.e., the HDR pathway. The S-RNH202 expression renders cells more dependent on HDR, as the accumulated rNMPs are being actively hydrolyzed by RNase H2 activity, whereas the rNMPs in the RNase H2 deletion strains subject to spontaneous hydrolysis, a less frequent occurrence. The SGA screen and subsequent validation identified 17 candidate genes linked to DNA metabolic processes, including DNA resection, HDR, and repair intermediate resolution, that may be involved in repair of rNMP-derived gDNA lesions in S phase. Rtt101 acts in a genetic pathway with Rad51 to promote rNMP repair Genetic evidence points to a crucial role of the Rtt101 Mms1-Mms22 ubiquitin ligase complex in the regulation of DNA repair and chromatin establishment [17] , [18] , [19] , [20] , [21] . These studies addressed the role of Rtt101 in the presence of exogenously induced DNA damage such as the Top1 poison camptothecin (CPT), the alkylating agent methylmethanesulfonate (MMS), or the ribonucleotide reductase inhibitor hydroxyurea (HU). Here, we found that Rtt101and the adaptor subunit Mms1 are also required when endogenous DNA lesions at genomic rNMP arise in S phase (Fig. 1G ). MMS22 , a member of the complex, was not a hit in the screen but was manually confirmed thereafter (Fig. 2A ). Fig. 2: Rtt101, histone modifiers and HDR factors promote cell viability when genomic rNMPs are hydrolyzed in S phase. A Tetrads from Rtt101 Mms1-Mms22 complex-deficient diploid strains in combination with S-RNH202-TAP revealed smaller colony sizes (colonies in circles). The genetic suppressor of rtt101 Δ, mrc1 Δ is sufficient to fully reverse the growth phenotype [19] (colonies in squares). B Tetrads from dissections of Rtt101 Mms1-Mms22 complex-deficient diploid strains in the S-RNH202-TAP pol2-M644G genetic background augmented the sickness. The rtt101 Δ S-RNH202-TAP pol2-M644G lethality was less penetrant compared to the mms1 Δ and mms22 Δ mutants, but after propagating, these small colonies were mostly inviable or acquired suppressor mutations. C Tetrad dissections of rad52 Δ with RNH202-TAP cell cycle alleles demonstrates that the S-RNH202-TAP rad52 Δ double mutant is inviable. D The phenotype from ( C ) was exacerbated when increasing the rNMP load ( pol2-M644G ). E The tetrads for RAD51 deletion with all cell cycle alleles of RNH202 shows that the S-RNH202 rad51 Δ double mutant is sick but viable. F Spot assay shows epistasis between S-RNH202-TAP rtt101 Δ and S-RNH202-TAP rad51 Δ double mutants and the S-RNH202-TAP rtt101 Δ rad51 Δ triple mutant. G Alkaline gel electrophoresis of the genotypes used in F) showed epistasis in terms of gDNA fragmentation between S-RNH202-TAP rtt101 Δ and S-RNH202-TAP rad51 Δ double mutant and the S-RNH202-TAP rtt101 Δ rad51 Δ triple mutant (compare lanes 3, 4, 5). The neutral gel serves as control for gDNA purity and integrity. Two alkaline gels revealed the same result. H Western blot analysis of checkpoint status by phospho-shift analysis of Rad53. The DNA profiles showed a 2n peak accumulation in line with the activated Rad53 checkpoint. I Viability analysis of exponential cultures stained with SYTOX Green shown as Scatter dot blot (line = mean, error bars = SD). “Boil” is the boiled positive control representing 100% dead hence SYTOX green positive cells. The unstained wild type sample serves as background control. Statistical analysis with GraphPadPrism8 (multiple comparison ANOVA test), n = 2 for all samples except rnh201 Δ rtt101 Δ and S-RNH202-TAP rtt101 Δ n = 4 samples. Source data are provided as a Source Data file. Full size image Consistent with the entire Rtt101 Mms1-Mms22 complex being important for rNMP tolerance, the individual deletions of RTT101 , MMS1 , and MMS22 are all compromised for growth in combination with S-RNH202 (Fig. 2A ). While colony growth is mildly affected in rtt101 Δ S-RNH202 , the deletion of MMS1 and MMS22 results in stronger effects (Fig. 2A , circled colonies). Increasing the rNMP load 10-fold using the pol2-M644G allele augments the synthetic sickness of S-RNH202 expression in Rtt101 complex mutants (Fig. 2B ). Although small spores form initially, they eventually become enviable, indicating the presence of severe genomic instability in these strains. The RNase H2 enzyme contains a C-terminal PIP box motif that mediates binding to proliferating cell nuclear antigen (PCNA), which enhances RNase H2 processivity in vitro [22] . The PIP box motif in RNase H2 is not required to produce the synthetic sick genetic interaction between rtt101 Δ and S-RNH202 (Supplementary Fig. 2F, G ), suggesting PIP box independent toxicity. The fork protection protein and checkpoint regulator Mrc1 is a genetic suppressor of MMS and CPT-sensitivity in rtt101 Δ cells [19] . Noteworthy, mrc1 Δ was also sufficient to rescue the growth of Rtt101 Mms1-Mms22 deficient S-RNH202 strains (Fig. 2A ). We are following up the underlying mechanism as to why mrc1 Δ rescues this phenotype, which will be described elsewhere. We tested the notion that Top1 may be responsible for the synthetic sick interaction of S-RNH202 and rtt101 Δ. Since the rtt101 Δ S-RNH202 pol2-M644G mutant is inviable (Fig. 2B ), we switched to HU instead of pol2-M644G to modulate the genomic rNMP load. HU has been previously shown to increase the genomic rNMP load in yeast and mammalian cells [23] , [24] . As expected, in the presence of HU, the S-RNH202 allele was synthetic sick with rtt101 Δ (Supplementary Fig. 3A ). Although the Top1-mediated RER-backup pathway can be mutagenic and accounts for cellular toxicity in absence of RNase H2 [10] , the synthetic sickness of rtt101 Δ S-RNH202 was Top1-independent (Supplementary Fig. 3B ). Moreover, the overexpression of RNase H1 did not improve growth in the rtt101 Δ S-RNH202 strains, suggesting that the toxicity is R-loop independent (Supplementary Fig. 3C ). Finally, we combined the S-RNH202 allele with the RER-deficient rnh201-RED allele, a separation of function mutant of RNase H2 ( [13] , reviewed in [25] ), that is RER defective, but can still remove R-loops, to show that hydrolyzed rNMPs in S phase require Rtt101 (Supplementary Fig. 3D, E ). The spot assay and the liquid growth assay data solidify that the rtt101 Δ S-RNH202 double mutant has reduced viability due to the RNase H2 ribonucleotide excision activity in S phase as the rtt101 Δ S-RNH202 RNH201 mutant is sicker and has longer population doubling time compared to the rtt101 Δ S-RNH202 rnh201 Δ mutant and the rtt101 Δ S-RNH202 rnh201-RED strain (Supplementary Fig. 3D, E ). Together, we showed that the role of Rtt101 in cells with high rNMP load and RNase H2 dysfunction is independent of Top1 and R-loops and dependent on the hydrolysis of genomic rNMPs by, for example the S-phase restricted RNase H2 allele. To test if Rtt101 and other HDR genes promote the repair of genomic rNMPs and their lesions, we performed genetic epistasis experiments combined with alkaline gel electrophoresis to monitor the genomic rNMP abundance in the presence and absence of the putative repair pathway. As previously demonstrated, the RAD52 gene becomes essential when rNMPs hydrolyze enzymatically through S-RNH202 (Fig. 2C ). This phenotype is exacerbated when the rNMP load is increased through pol2-M466G expression (Fig. 2D ). Expression of G1-RNH202 also slightly affects the growth of rad52 Δ cells, which again suggests that RNase H2 may be acting in G1, but some unrepaired nicks are carried into S phase (Fig. 2C ). Due to the lethality of RAD52 deletions in the S-RNH202 genetic background, we could not perform genetic epistasis experiments with loss of RTT101 . The rad51 Δ S-RNH202 double mutant, however, is growth impaired, yet viable (Fig. 2E ). Hence, we performed epistasis experiments comparing the loss of RTT101 and RAD51 and both genes together in the S-RNH202 background (Fig. 2F ). The rtt101 Δ rad51 Δ S-RNH202 triple mutant is not additive, suggesting that RTT101 and RAD51 may function in the same genetic pathway of rNMP-derived nick repair in S phase (Fig. 2F ). We employed alkaline gel electrophoresis to visualize the genomic rNMP load in rtt101 Δ and rad51 Δ strains in the presence of increased S phase rNMP-nicking ( S-RNH202 ). In addition to rNMP-hydrolysis activity in S phase, the S-RNH202 strain accumulates rNMPs (Fig. 2G , lane 1 compared to lane 2). Strikingly, the loss of either RTT101 or RAD51 alone, and in combination, resulted in higher DNA fragmentation in alkaline conditions and loss of the prominent genomic DNA band, indicative of fragmented genomic DNA, hence lack of rNMP repair (Fig. 2G , lanes 3, 4, 5 compared to 2, and quantification graph below). The rtt101 Δ strains show basal checkpoint activation visualized by phospho-Rad53 analysis (Fig. 2H ). In line with the elevated rNMP load and non-repaired DNA damage leading to impaired viability, the rtt101 Δ S-RNH202 mutants have fully activated the Rad53-checkpoint (Fig. 2H ). In addition, we observed 4% cell death in that population without further challenge (Fig. 2I ). This supports the idea of a repair pathway as loss of the repair factors, Rtt101 and Rad51, result in a repair defect accompanied by an activated DNA damage checkpoint, hence the failure to efficiently remove rNMPs. Epistasis between rtt101 Δ and rad51 Δ in S-RNH202 -cells was also confirmed by DNA damage checkpoint activation (Supplementary Fig. 3F, G ) and by population doubling time measurement in liquid cultures (Supplementary Fig. 3H ). Together, these data demonstrate that the Rtt101 complex works together with the recombination machinery to repair rNMPs, and not R-loops, that get nicked in the S phase. Rtt101 becomes essential in S phase to overcome Top1-independent rNMP-derived toxicity We have demonstrated that the S-RNH202 allele is very similar to the RNase H2 deletion (Supplementary Fig. 1A–C ), hence we predicted that RTT101 would also play an important role in the S phase repair of hydrolyzed rNMPs in RER-deficient strains. Indeed, the rtt101 Δ rnh201 Δ double mutants were sensitive to HU as compared to the respective single mutants (Fig. 3A ). Importantly, RNH1 overexpression, which reduces R-loop levels, did not rescue the rtt101 Δ rnh201 Δ viability defect in the presence of HU (Fig. 3A ), suggesting that R-loops may not be responsible for the growth defects. As RNase H2 has a dual role in RNA-DNA hybrid removal, and participates in R-loop removal [7] , [26] , we again employed the rnh201-RED allele that retains R-loop removal activity but fully lacks RER-activity [13] . We found that the RER-proficient RNH201 wild type allele could rescue the growth defect of rtt101 Δ rnh201 Δ mutants in the presence of HU; however, strains expressing the rnh201-RED allele were as sick as the vector control (Fig. 3B ). This confirmed that persisting genomic rNMPs are the underlying cause of the slow growth in rtt101 Δ rnh201 Δ cells (Fig. 3 A, B ). The rtt101 Δ rnh201 Δ pol2-M644G triple mutant was genetically unstable, therefore we employed an RNH201-AID* auxin-inducible degron [27] , to highly reduce RNase H2 activity in the presence of auxin (Supplementary Fig. 4A, B ). Similar to the rtt101 Δ rnh201 Δ double mutant, rtt101 Δ RNH201-AID* cells presented a mild growth defect upon exposure to auxin (Fig. 3C ). 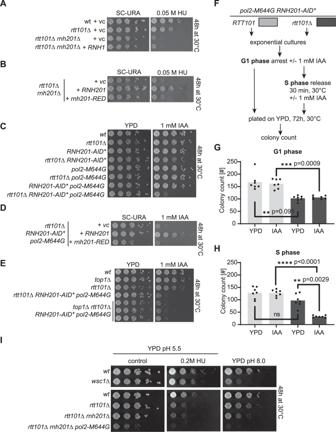Fig. 3: Rtt101 becomes essential in S phase in a Top1-independent manner to overcome rNMP-derived toxicity. AThertt101Δrnh201Δ double mutant is synthetic lethal in the presence of HU (hydroxyurea). Transformation withRNH1did not affect the growth of the double mutant on HU-containing agar plates.BTransformation withRNH201did rescue growth of thertt101Δrnh201Δ double mutant on HU plates, while the RER-deficient separation-of-functionrnh201-REDmutant had no effect. Two independent transformants of each genotype showed the same result.CDepletion ofRNH201-AID*in the presence of IAA (auxin) resulted in a synthetic sick growth phenotype withrtt101Δ, which was amplified into a synthetic lethal phenotype when combined withpol2-M644G.DComplementation of thepol2-M644G rtt101ΔRNH201-AID* triple mutant with wild typeRNH201rescued growth on auxin plates, while thernh201-REDmutant did have no effect.EThe synthetic lethality of thepol2-M644G rtt101ΔRNH201-AID*triple mutant on auxin plates was Top1-independent. Three independent strains from separate tetrads were spotted to confirm Top1-independence of the observed phenotype.F–HLiquid cultures with the indicated genotypes were synchronized with α-factor in the G1 phase in the presence of IAA to depleteRNH201-AID*. The arrested cultures were either directly plated on YPD agar plates (colony count panelG), or released into the S phase in the presence of IAA, followed by plating on YPD agar plates (colony count panel H). Scatter dot blot with bar at mean fromn= 7 plate counts per genotype and condition. Statistics were performed with GraphPad Prism8 (multiple comparison ANOVA).IThe spot assay withrtt101Δ strains in the RER-deficientrnh201Δ and the rNMP accumulatingpol2-M644Gbackground revealed that alkalization of the YPD agar was sufficient to phenocopy the synthetic sick growth defects seen in the presence of HU. Source data are provided as a Source Data file. Upon addition of the pol2-M644G allele to increase the genomic rNMP load, the rtt101 Δ RNH201-AID* pol2-M644G triple mutant was inviable in the presence of auxin (Fig. 3C ). The rnh201-RED allele could not rescue the synthetic lethality of the rtt101 Δ RNH201-AID* pol2-M644G triple mutants in the presence of auxin (Fig. 3D ). 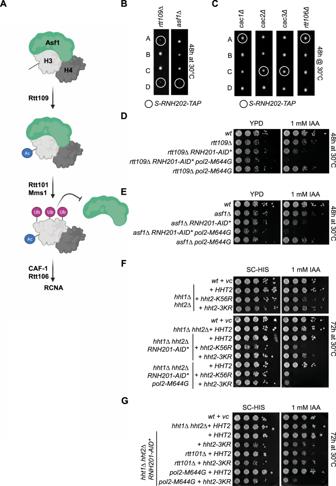Fig. 4: Rtt101 mediates the repair of rNMP-derived DNA damage in S phase through histone H3 ubiquitylation. AScheme of the contribution of the histone chaperone Asf1, the histone acetyl transferase Rtt109 and the ubiquitin ligase Rtt101Mms1to the replication-coupled nucleosome assembly (RCNA) pathway. Sequence of events (modified from ref.20): Asf1 binds tode novosynthesized H3-H4 dimers and Rtt109 acetylates H3 followed by ubiquitylation of H3 through Rtt101 that lead to the release of Asf1 and facilitates DNA incorporation. Note that an acetylation deficientH3-K56Rmutant is reminiscent ofRTT109deletion and an ubiquitylation-deficientH3-3KRmutant is reminiscent of theRTT101deletion. Created with BioRender.com.BManual tetrad dissection confirmed the synthetic lethal phenotype between theS-RNH202allele and the histone remodeler genesRTT109andASF1(double mutant colonies in circles).CRepresentative tetrads from single CAF-1 complex deletion mutants (cac1Δ,cac2Δ,cac3Δ) in combination withS-RNH202-TAPto check contribution of the RCNA pathway. Note that these genes work redundantly and they are synthetic lethal with each other, hence we cannot exclude their contribution.DSpot assays withRTT109deletion mutants shows that loss ofRTT109is toxic in RER-deficient strains with high rNMP load (pol2-M644G).EThe same is true for loss of the histone chaperoneASF1.FSpot assays with histone H3 mutants deficient for Lysine-56 acetylation (“H3-K56R”) and Rtt101-dependent Lysine-121,122,125 triple ubiquitylation (“H3-3KR”)20. These plasmid-borne mutant versions of histone H3 replaced the two H3 coding genes (HHT1andHHT2)that were deleted from the genome (see yeast strain list for the respective complete genotypes). Histone H3 Lysine-56 acetylation became essential in RER-deficient cells (RNH201-AID*on IAA plates). TheH3-3KRstrain revealed mild sickness in RER-deficient cells but was inviable when rNMP levels increased with thepol2-M644Gallele.GStrains from (F) were combined withRTT101deletion to confirm the epistasis betweenRTT101-deficiency and H3 ubiquitylation deficiency (compare lanes 4–6). 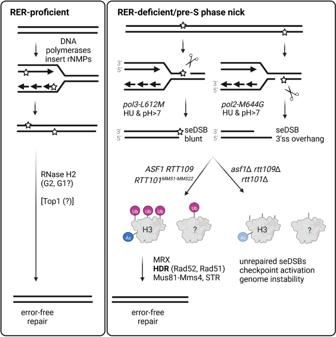Fig. 5: Top1-independent NLR pathway is essential when rNMPs cause pre-S phase nicks that result in seDSB. DNA polymerases transiently incorporate single rNMPs into the genome during replication and repair. The RER pathway removes genomic rNMPs immediately in the subsequent G2 phase. In RER-deficient, or RER-dysfunctional cells the Top1-mediated backup pathway deals with rNMP-removal. However, if high amounts of persistent genomic rNMPs accumulate in RER-deficient, or RER-dysfunctional cells, the likelihood increases that hydrolysis-prone rNMPs form ssDNA nicks. When the replication fork encounters such an rNMP-derived nick, a toxic seDSB is formed. End topology of the seDSB may differ dependent on the location of the nick39. To repair the rNMP-derived seDSB lesions, functional RCNA is required. The histone remodelers Asf1 and Rtt109 act upstream of Rtt101Mms1-Mms22, presumably accompanied by the resection of the seDSB by MRX (Mre11-Rad50-Xrs2), followed by HDR (Rad52, Rad51) and resolution of the HDR intermediates (Mus81-Mms4, Sgs1-Top3-Rmi1) to result in the error-free repair of the seDSB. InRTT101-deficient cells with high rNMP load, histone H3 does not become ubiquitylated and downstream error-free HDR repair of the seDSB is compromised causing genomic instability likely by alternative, error-prone repair attempts. Abbreviations: NLR rNMP-derived nick lesion repair, rNMP single ribonuclesoide monophates, RER ribonucleotide excision repair, seDSB single-ended double strand break, ssDNA single stranded DNA, RCNA replication-coupled nucleosome assembly, HDR homology-directed repair. Created with BioRender.com. The deletion of either MMS1 or MMS22 showed similar genetic interactions with RNase H2 impairment, suggestive of the entire E3 ubiquitin ligase complex being required to tolerate increased rNMP levels (Supplementary Figure 4C ). As with the S-RNH202 allele , we tested whether Top1-processing of ribonucleotides was responsible for the phenotype of rtt101 Δ RNH201-AID* pol2-M644G cells. In line with the S-RNH202 allele (Supplementary Fig. 3B ), the deletion of TOP1 did not rescue the viability of rtt101 Δ RNH201-AID* pol2-M644G in the presence of auxin (Fig. 3E ). The inability of top1 Δ to rescue the phenotype was consistent for the entire Rtt101 Mms1-Mms22 complex (Supplementary Figure 4D ). As we previously demonstrated that RTT101 acts in the same pathway as HDR for survival with S-RNH202 expression, we also expected that defective RER would lead to a fitness disadvantage when HDR was inactive. To this end, we observed that the loss of RAD52 was defective for growth in the presence of the rnh201-RED allele (Supplementary Fig. 4E ) . The viability of a RER-deficient pol2-M644G strain fully relied on the presence of RAD52 , furthermore indicating that the lesion potential correlates directly with the amount of rNMPs (Supplementary Fig. 4F ). Together, these results are consistent with an Rtt101-mediated HDR being required to repair nicked rNMPs in S phase, independent of Top1 mediated cleavage. Fig. 3: Rtt101 becomes essential in S phase in a Top1-independent manner to overcome rNMP-derived toxicity. A The rtt101 Δ rnh201 Δ double mutant is synthetic lethal in the presence of HU (hydroxyurea). Transformation with RNH1 did not affect the growth of the double mutant on HU-containing agar plates. B Transformation with RNH201 did rescue growth of the rtt101 Δ rnh201 Δ double mutant on HU plates, while the RER-deficient separation-of-function rnh201-RED mutant had no effect. Two independent transformants of each genotype showed the same result. C Depletion of RNH201-AID* in the presence of IAA (auxin) resulted in a synthetic sick growth phenotype with rtt101 Δ, which was amplified into a synthetic lethal phenotype when combined with pol2-M644G . D Complementation of the pol2-M644G rtt101 Δ RNH201-AID * triple mutant with wild type RNH201 rescued growth on auxin plates, while the rnh201-RED mutant did have no effect. E The synthetic lethality of the pol2-M644G rtt101 Δ RNH201-AID* triple mutant on auxin plates was Top1-independent. Three independent strains from separate tetrads were spotted to confirm Top1-independence of the observed phenotype. F – H Liquid cultures with the indicated genotypes were synchronized with α-factor in the G1 phase in the presence of IAA to deplete RNH201-AID* . The arrested cultures were either directly plated on YPD agar plates (colony count panel G ), or released into the S phase in the presence of IAA, followed by plating on YPD agar plates (colony count panel H). Scatter dot blot with bar at mean from n = 7 plate counts per genotype and condition. Statistics were performed with GraphPad Prism8 (multiple comparison ANOVA). I The spot assay with rtt101 Δ strains in the RER-deficient rnh201 Δ and the rNMP accumulating pol2-M644G background revealed that alkalization of the YPD agar was sufficient to phenocopy the synthetic sick growth defects seen in the presence of HU. Source data are provided as a Source Data file. Full size image The Rtt101 Mms1-Mms22 ubiquitin ligase complex is associated with the replisome during S phase [19] and becomes essential when rNMPs are hydrolyzed in S phase by S-RNH202 (Figs. 1 , 2 ). We wanted to test if rNMP-derived damage in a single S phase requires the immediate activity of Rtt101 Mms1-Mms22 . Therefore, we performed a colony formation assay to assess cell viability when rNMP removal is prevented either in the G1 phase or during S phase (Fig. 3F–H and Supplementary Fig. 4G, H ). We arrested RNH201-AID* pol2-M644G and rtt101 Δ RNH201-AID* pol2-M644G cultures in the G1 phase in the presence of auxin to degrade Rnh201 and prevent RNase H2 activity. To assess the toxicity of rNMP accumulation in G1 phase, we plated the cultures directly on rich medium and quantified the number of colonies formed (Fig. 3 G). Alternatively, the synchronized cultures were released from the G1 arrest into the S phase still in the presence of auxin to abolish RNase H2 activity during S phase entry and progression. S phase cultures were also plated on rich medium, thereby allowing the re-accumulation of RNase H2 (Fig. 3H ). We monitored the cell cycle phases of the cultures by flow cytometry (Supplementary Fig. 4H ). We observed an overall 20% viability reduction in the rtt101 Δ background (Fig. 3 G, H ). RER-deficiency did not affect the cell viability during G1 phase (Fig. 3G , compare dark grey columns). However, in the absence of Rtt101 there was a 70% reduction in cell viability when RER-deficient cells progressed through S phase (Fig. 3H , compare dark grey columns). Therefore, non-repaired rNMPs are only toxic in rtt101 Δ cells in the S phase of the cell cycle, and not in G1. The 2′-hydroxyl group renders rNMPs susceptible to spontaneously hydrolyze the phosphodiester backbone compared to the more stable and resistant DNA deoxy sugars. Since this hydrolysis reaction is more likely in a basic environment, we assumed that growth in alkaline conditions may increase the likelihood that hydrolysis at genomic rNMPs will occur. Alkaline conditions were therefore expected to impact the growth of rtt101 Δ strains similar as the presence of hydroxyurea or the absence of RER. Saccharomyces cerevisiae media (YPD) has pH5.5 and therefore is mildly acidic. We increased the pH of solid agar medium to pH8.0. We confirmed alkaline pH8.0 in agar plates by using the wsc1 Δ strain that renders cells sensitive to alkali pH stress [28] (Fig. 3I ). The rtt101 Δ strain was mildly sensitive to pH8.0 whereas rtt101 Δ rnh201 Δ cells were highly sensitive to alkaline conditions (Fig. 3I ). The unstable rtt101 Δ rnh201 Δ pol2-M644G triple mutant was fully inviable on pH8.0 (Fig. 3I ). So far we utilized hydroxyurea (HU) or the leading strand mutator pol2-M644G to elevate genomic rNMP levels. As the SGA screen (Fig. 1 ) was performed in presence of the wild type polymerase alleles POL3 and POL2 we anticipate that the rNMP-derived lesions in the S-RNH202 strain should occur randomly in the genome. Indeed, the pol3-L612M allele recapitulated the negative synthetic effects in RER-deficient and S phase restricted RNase H2 conditions in the absence of RTT101 (Supplementary Fig. 5A–C ). Compared to pol2-M644G, the pol3-L612M effects were milder, which would be in line with the lower rNMP incorporation rate of POL3 compared to POL2 [12] . Interestingly, we noticed a synthetic sick interaction between rtt101 and pol3-L612M in the presence of high HU (Supplementary Fig. 5C, D ). In conclusion, both mutator alleles boost genomic rNMP levels and enhance the rNMP-derived negative synthetic sick genetic interactions between RNase H2 dysfunction and RTT101 . In summary, we report that the negative genetic interaction between the deletion of Rtt101 Mms1-Mms22 ubiquitin ligase subunits and RNase H2 defects is due to RER-deficiency and is exacerbated in rNMP accumulating ( pol2-M644G , HU) condition. In RER-defective cells, rNMPs are likely hydrolyzed prior to, or during, S phase and require Rtt101 mediated HDR for repair upon encounter with the replisome. In line with the physical association with the replisome in S phase [19] , Rtt101 function is essential during S phase to counteract rNMP-derived cellular toxicity. Rtt101 may drive rNMP repair in S phase through histone H3 ubiquitylation Using different genetic models ( S-RNH202 allele, RNase H2 deletion, alkaline conditions, pol2-M644G allele, rnh201-RED allele), we demonstrated that the Rtt101 Mms1-Mms22 ubiquitin ligase complex is required to deal with Top1-independent rNMP-derived DNA damage in S phase. We speculate that we may have found the genetic requirements for a unique rNMP-derived lesion repair pathway that acts in S phase, complementing the RER and the Top1 pathways [14] . We set out to get a deeper molecular understanding by further probing the genetic interactions from the S-RNH202 SGA genetic network (Fig. 1 ) and potentially identify substrates for Rtt101. The Rtt101 Mms1-Mms22 complex has previously been shown to ubiquitylate histone H3 on three lysine (K) residues (K121, K122, and K125) [20] . The modification does not lead to proteasomal degradation, but rather facilitates the deposition of newly synthesized histones during replication-coupled nucleosome assembly (RCNA). Other, non-replication related, substrates of Rtt101 Mms1-Mms22 have been reported in yeast [29] , whereas multiple targets of Cul4 have been elucidated in human cells [30] , [31] , [32] , [33] , [34] , [35] . The histone chaperone Asf1 and the histone acetylase Rtt109, which acetylate lysine 56 of H3 (H3K56), act upstream of Rtt101 Mms1-Mms22 in terms of nucleosome assembly [20] (Fig. 4A ). Similar to RTT101 , the ASF1 and RTT109 genes were essential for cellular survival when rNMPs were nicked in the S phase (Fig. 4B ). In the RCNA pathway, Rtt101 is responsible for the ubiquitylation of newly synthesized histone H3 on three lysine residues, which release the H3-H4 dimer from the histone chaperone Asf1 (Fig. 4A ). As the downstream RCNA factors CAC1/RLF2 , CAC2 , CAC3/MSI1 that form the CAF-1 complex and RTT106 have redundant roles [36] , the single deletions do not affect S-RNH202 colony growth (Fig. 4C ). CAF-1 deletion combined with RTT106 deletion is synthetic lethal, which is why we cannot rule out their contribution. We generated heterozygous diploid strains and derived the haploid double mutants to test the impact of Rtt109 and Asf1 loss in a RER-deficient condition using the RNH201-AID* degron and the pol2-M644G allele (Fig. 4 D, E ). Strikingly, triple mutants displayed lethality in the presence of auxin, reflecting the major role of RCNA factors, Asf1 and Rtt109, in the repair of rNMP-derived lesions (Fig. 4 D, E ). Fig. 4: Rtt101 mediates the repair of rNMP-derived DNA damage in S phase through histone H3 ubiquitylation. A Scheme of the contribution of the histone chaperone Asf1, the histone acetyl transferase Rtt109 and the ubiquitin ligase Rtt101 Mms1 to the replication-coupled nucleosome assembly (RCNA) pathway. Sequence of events (modified from ref. [20] ): Asf1 binds to de novo synthesized H3-H4 dimers and Rtt109 acetylates H3 followed by ubiquitylation of H3 through Rtt101 that lead to the release of Asf1 and facilitates DNA incorporation. Note that an acetylation deficient H3-K56R mutant is reminiscent of RTT109 deletion and an ubiquitylation-deficient H3- 3KR mutant is reminiscent of the RTT101 deletion. Created with BioRender.com. B Manual tetrad dissection confirmed the synthetic lethal phenotype between the S-RNH202 allele and the histone remodeler genes RTT109 and ASF1 (double mutant colonies in circles). C Representative tetrads from single CAF-1 complex deletion mutants ( cac1 Δ, cac2 Δ, cac3 Δ) in combination with S-RNH202-TAP to check contribution of the RCNA pathway. Note that these genes work redundantly and they are synthetic lethal with each other, hence we cannot exclude their contribution. D Spot assays with RTT109 deletion mutants shows that loss of RTT109 is toxic in RER-deficient strains with high rNMP load ( pol2-M644G ). E The same is true for loss of the histone chaperone ASF1 . F Spot assays with histone H3 mutants deficient for Lysine-56 acetylation (“ H3-K56R ”) and Rtt101-dependent Lysine-121,122,125 triple ubiquitylation (“ H3-3KR ”) [20] . These plasmid-borne mutant versions of histone H3 replaced the two H3 coding genes ( HHT1 and HHT2) that were deleted from the genome (see yeast strain list for the respective complete genotypes). Histone H3 Lysine-56 acetylation became essential in RER-deficient cells ( RNH201-AID* on IAA plates). The H3-3KR strain revealed mild sickness in RER-deficient cells but was inviable when rNMP levels increased with the pol2-M644G allele. G Strains from ( F ) were combined with RTT101 deletion to confirm the epistasis between RTT101 -deficiency and H3 ubiquitylation deficiency (compare lanes 4–6). Full size image To assess if the Rtt101-dependent H3 ubiquitylation has a direct role in rNMP-lesion repair, we combined the ubiquitylation-deficient H3-3KR mutant [20] with an RER-deficient background using the RNH201-AID* degron (Fig. 4F ). Rtt109-mediated H3-K56 acetylation occurs upstream of Rtt101-dependent H3 ubiquitylation [20] . The H3-K56R acetylation-deficient strain was synthetic sick with loss of RNase H2 and inviable when rNMPs accumulate in the RNH201-AID* pol2-M644G strain background (Fig. 4F ). Interestingly, the H3-3KR ubiquitylation-deficient mutant could support growth upon loss of RNase H2 better than the H3-K56R mutant, however, Rtt101-dependent H3-ubiquitylation became essential when rNMP load increased in the RNH201-AID* pol2-M644G strain (Fig. 4F ). To show that Rtt101 and the Rtt101-dependent H3 ubiquitylation behave in an epistatic manner, we deleted RTT101 in the H3-3KR mutant strains. Indeed, deleting RTT101 , or impairing H3 ubiquitylation ( H3-3KR ), or the combination of both impaired cell viability to the same degree in RER-deficient strains (Fig. 4G ). This suggests that histone H3 is a key target of Rtt101, and we conclude that Rtt101 Mms1-Mms22 dependent histone H3 ubiquitylation at lysines-121, -122, and -125 is critical for the repair of rNMP-derived DNA damage. However, it also suggests that other functions of the RCNA pathway may be important for rNMP repair in RER defective strains. Interestingly, Asf1 has a role in the regulation of Rad53 checkpoint control [37] . It will be important to unravel the unknown connections that still exist between Rtt101, DNA repair, checkpoint recovery, and chromatin (RCNA). Eukaryotic cells repair genomic rNMPs by RNase H2-initiated ribonucleotide excision repair (RER). The loss of RNase H2 function leads to the accumulation of genomic rNMPs, which then become, to an extent, substrates for error-prone repair by Top1 (reviewed in [14] ). Recently, it has been demonstrated that some human cancers harbour RNase H2 mutations, resulting in rNMP accumulation and Top1-mediated genome instability [6] . These cancers are considered “druggable” as Top1 lesions recruit PARP to sites of damage and hence become susceptible to PARP inhibitors [6] . Elucidating alternative rNMP repair pathways may yield additional factors and pathways that could potentially be targeted in RER defective human cancer cells. Importantly, it has been shown that RER-defective budding yeast have a nearly identical mutagenic signature profile as RER defective cancer cells [11] , hence making yeast a highly relevant model for the study of rNMP repair. The loss of RAD52 becomes essential in RER-defective yeast cells and TOP1 deletion can only partially rescue the loss of fitness, indicating that there might be additional sources for rNMP-mediated genome instability apart from Top1 [8] , [38] . Genomic rNMPs are prone to hydrolysis and nick formation and it was shown recently that the CMG helicase will eventually run off the DNA, if the leading strand template is nicked upstream of the replication fork [39] . Hence, we hypothesized that the HDR machinery was repairing rNMP-induced lesions (seDSB) that occur when a nicked rNMP encounters replication [8] . In support of this idea, increased rNMP-nicking in RER-deficient cells rendered cells dependent on HDR, independent of Top1 [8] . Here, we employed the S-RNH202 allele to induce seDSBs at rNMPs to look for mutants with reduced fitness similar to rad52 Δ, in a genome-wide screening approach (Fig. 1 ). As a result, we elucidated a genetic network for rNMP-derived n ick l esion r epair (NLR) (Fig. 5 ). NLR includes the Rtt101 ubiquitin ligase, the Rad52-based HDR machinery, the MRX (Mre11-Rad50-Xrs2) complex, and the Rtt109/Asf1 replication-coupled nucleosome assembly (RCNA) pathway (Fig. 1 ). In addition, we found the STR (Sgs1-Top3-Rmi1) and Mus81-Mms4 complexes, which likely provide resolution of the multiple recombination intermediates formed during HDR [40] (Fig. 1 ). We showed that the exclusive nicking of rNMPs in S phase is particularly toxic in rtt101 Δ cells (Fig. 2A ). Indeed, we could demonstrate that loss of RAD51 and RTT101 are epistatic in terms of rNMP repair (Fig. 2G ). Furthermore, we confirmed that loss of RTT101 was sufficient to kill RER-deficient cells in a Top1-independent manner (Fig. 3E ). We were also able to conclude that Rtt101 function is required in S phase (Fig. 3H ), which is in alignment with its replisome association [19] . Moreover, the mutated allele of histone H3 that can no longer be ubiquitylated by Rtt101 (H3-3KR) also renders cells highly sensitive to high levels of rNMPs (Fig. 4F–G ). Although Rtt101, HDR and H3 ubiquitylation are all working together in a genetic pathway it remains unclear as to how Rtt101 promotes HDR. Fig. 5: Top1-independent NLR pathway is essential when rNMPs cause pre-S phase nicks that result in seDSB. DNA polymerases transiently incorporate single rNMPs into the genome during replication and repair. The RER pathway removes genomic rNMPs immediately in the subsequent G2 phase. In RER-deficient, or RER-dysfunctional cells the Top1-mediated backup pathway deals with rNMP-removal. However, if high amounts of persistent genomic rNMPs accumulate in RER-deficient, or RER-dysfunctional cells, the likelihood increases that hydrolysis-prone rNMPs form ssDNA nicks. When the replication fork encounters such an rNMP-derived nick, a toxic seDSB is formed. End topology of the seDSB may differ dependent on the location of the nick [39] . To repair the rNMP-derived seDSB lesions, functional RCNA is required. The histone remodelers Asf1 and Rtt109 act upstream of Rtt101 Mms1-Mms22 , presumably accompanied by the resection of the seDSB by MRX (Mre11-Rad50-Xrs2), followed by HDR (Rad52, Rad51) and resolution of the HDR intermediates (Mus81-Mms4, Sgs1-Top3-Rmi1) to result in the error-free repair of the seDSB. In RTT101 -deficient cells with high rNMP load, histone H3 does not become ubiquitylated and downstream error-free HDR repair of the seDSB is compromised causing genomic instability likely by alternative, error-prone repair attempts. Abbreviations: NLR rNMP-derived nick lesion repair, rNMP single ribonuclesoide monophates, RER ribonucleotide excision repair, seDSB single-ended double strand break, ssDNA single stranded DNA, RCNA replication-coupled nucleosome assembly, HDR homology-directed repair. Created with BioRender.com. Full size image One possibility would be that rNMPs are more susceptible to induce nicks because the chromatin structure of rtt101 Δ cells is altered due to the RCNA defects. This would be consistent with decreased nucleosome deposition and a more open chromatin state. In agreement, it has been reported that telomeric heterochromatin is lost in rtt101 Δ and mms1 Δ mutants [21] . It will be important determine if hydrolyzed rNMPs are more frequent in more accessible chromatin environments and if such environments actually increase in the absence of the Rtt101 complex. Alternatively, it could be that Rtt101-mediated H3 modifications are important for the HDR reaction itself. This hypothesis is supported by the fact that deletion of the fork protection protein and damage checkpoint mediator MRC1 can rescue the sensitivity of rtt101 Δ cells to genotoxic agents [19] as well as to accumulation of rNMPs (Fig. 2A ). Indeed, Mrc1 can differentially regulate resection and HDR at DSBs [41] and it was recently demonstrated that this involves changes in chromatin compaction [42] . Further support that the repair of rNMP-derived lesions is coupled to alterations of chromatin was shown in a recent study in human cells [43] . Specifically, they looked at seDSB damage caused by the replisome running into Top1-DNA adducts after CPT treatment. In line with our yeast genetic network, HDR factors, MRN, RAD51, and MMS22L-TONSL were found to be associated with the broken forks in human cells [43] . Interestingly, these broken and stalled replication forks presented a distinct chromatin environment with a defect in histone deposition [43] . In addition, sister chromatin cohesion is important at seDSBs to ensure that repair occurs primarily from the sister chromatid and not a homologous chromosome. Rtt101, Mms1, and Mms22 promote sister chromatid cohesion through their replisome association [44] . Interestingly, the cohesion-like Smc5/6 complex becomes essential in the absence of RER ( [45] ) and may also be intertwined with the Rtt101, Rtt109, HDR-mediated repair of rNMPs. In fission yeast, the mega-nuclease complex MRN (Mre11-Rad50-Nbs1) is critical to control sister chromatid cohesion at replication-associated seDSBs to allow HDR repair and prevent Ku-mediated DSB repair [46] . In accordance, all subunits of the Saccharomyces cerevisiae MRX complex seem to be essential for NLR (Supplementary Fig. 1I ). The restriction to the 4790 non-essential genes, covering 75% of the total 6275 S. cerevisiae ORFs, is one important limitation of this study. However, the comparative analysis to a published dataset including essential genes allowed us to pinpoint the NSE4 gene, a subunit of the Smc5/6 complex as a factor relevant for NLR (Supplementary Fig. 2E ). Since cohesin and cohesin-like factor are essential, they were not revealed in our screen and will have to be systematically tested using conditional alleles. Our current working model integrates the NLR network into a repair pathway occurring after a nicked DNA template would lead to the formation of a seDSB during replication (Fig. 5 ). According to recent in vitro work using Xenopus laevis extracts, the fate of a replication fork encountering a nicked DNA template is the formation of a seDSBs both with a leading strand template nick and a lagging strand template nick [39] . Through the use of polymerase mutants that incorporated rNMPs in a strand specific manner, we determined that the Rtt101 E3 ligase became essential at rNMPs in a strand independent manner. It will be important to determine whether the Rtt101 E3 human equivalent, Cullin-Ring-Ligase 4 (CRL4), also contributes to rNMP repair in RNase H2 defective cells, as this may represent alternative therapeutic opportunities, in addition to PARP inhibitors in RER defective cancer cells. It is feasible to put this to the test in the future as the CRL neddylation inhibitor MLN4924 was extensively studied and went into clinical trials for cancer intervention [47] , [48] . In this respect, it is interesting that the cullin subunit of CRL4 (CUL4A) is overexpressed in many human cancers [49] . The cancer-specific overexpression is a result of the genomic locus in human cells that undergoes amplification in cancers [50] . Hence, it is possible that this overexpression promotes CRL4-dependent DNA repair also in the context of other human deficiencies (e.g., RER). We speculate that the role for NLR could be greater than expected as the inside of a cancer cell is slightly alkaline (pH > 7), and could therefore promote rNMP-mediated hydrolysis of the DNA backbone. The intracellular alkalization of cancer cells seems connected to the initial oncogenic transformation and the progression of the tumour [51] , [52] . Translational studies will show if RER-defective human cancer cells with alkaline intracellular environment may even favour NLR due to augmented spontaneous rNMP hydrolysis. The NLR genes comprise DNA repair complexes that participate in a variety of well-characterized DNA repair pathways. However, in this combination, they have not been described elsewhere to our knowledge. Especially the connection of DNA repair (recombination, resection, unwinding) with chromatin remodelling (RCNA) is interesting and requires further study and careful separation of the multiple roles of e.g., MRX and STR complexes. Hence, we are favoring the idea that NLR could be relevant for the repair of all kinds of replisome-nick encounter-derived lesions in cycling cells with the common feature of a toxic seDSB as the damage site. Yeast strains and plasmids Saccharomyces cerevisiae strains used in this study derive of the standard S288C ( MATa his3 Δ 1 leu2 Δ 0 ura3 Δ 0 met15 Δ 0 ) strain and are listed in Supplementary Data 2 . Strains were grown under standard conditions in YPD (1% [w/v] yeast extract, 2% [w/v] peptone supplemented with 2% glucose) or in SC (0.2% [w/v] Synthetic Complete medium without specific amino acids, 1% [w/v] yeast nitrogen base supplemented with 2% glucose) at 30 °C if not indicated otherwise. Yeast transformations with plasmid or PCR products were performed with the standard lithium acetate polyethylene glycol (PEG) method [53] . Gene deletions, tagging, and generation of specific mutations were performed using standard PCR-based recombination methods and confirmation by sequencing. Plasmids and oligonucleotides are listed in Supplementary Data 3 . Yeast tetrad dissection For analysis of the meiotic product, we crossed a MATa with a MATalpha haploid strain, selected for diploids based on auxotrophy or antibiotic resistance, and patched the diploid strain on rich pre-Sporulation plates (YP agar with 6% [w/v] glucose]. Then we froze part of the patch and transferred part of the patch into Sporulation medium (1% potassium acetate, 0.005% zinc acetate buffer) and incubated the cultures with shaking at 23 °C. After a few days, the sporulation cultures were treated in a ratio of 1:1 [v/v] with Lyticase (L4020 Sigma Aldrich, 2.5 mg/ml, 200 units/µl, in 1 M D-Sorbitol) to digest the ascus. After 15–20 min at room temperature, the culture was applied to an agar plate and tetrads were dissected using a Singer micromanipulator. Colonies of haploid spores grew at 30 °C for three days. Images were taken at 48 and 72 h with the ChemiDoc™ Touch Imaging System (Bio-Rad). After three days, the spores were replica plated, genotypes were scored and strains were frozen in 15% glycerol-containing cryopreserved stocks at −80 °C. Strains are listed in Supplementary Data 2 . Flow cytometry analysis for DNA content Cells were fixed in 70% ethanol overnight and then treated with 0.25 mg/ml DNase- and Protease-free RNase A (ThermoFisher Scientific, 10753721) at 37 °C for 2 h and Proteinase K (Biofroxx, 1151ML010) at 50 °C for 2 h in 50 mM Tris-HCl pH7.5 buffer. The cell suspension was sonified using a Branson sonifier 450 for 5 s with output control 1 and duty cycle constant. Then, cells were stained with a final concentration of 2.4 µM SYTOX Green nucleic acid stain (ThermoFisher Scientific, 1076273). Measurement was performed on the BD LSRFortessa flow cytometer (BD Biosciences) using the BD FACSDiva software (v9.0.1). With low flow rate, 20,000 events were recorded. Analysis was performed with FlowJo (v10.8.0) using the following gating strategy: From the main population in FSC-A vs. SSC-A, doublets were excluded in the SYTOX Green A vs. W channel, and DNA content was assessed in the histogram of the SYTOX Green-A channel (Ex 488 nm, 530/30BP). Flow cytometry analysis for cell viability In contrast to measurements of the DNA content using ethanol-fixed dead cells, we collected exponentially growing cells and, without fixation, stained them with SYTOX Green to discriminate between living cells (do not take up SYTOX Green) and dead cells (will incorporate SYTOX Green). Cells were collected and the cell pellet was washed with 50 mM Tris pH 7.5 and resuspended in 1 ml 50 mM Tris pH 7.5 containing 0.5 μM SYTOX Green. Measurement and analysis were the same as for the DNA content analysis except for doublet exclusion, which was done in the SSC-A vs. W channel. As a control sample for dead cells, controls were incubated at 95 °C for 15 min and subjected to the described protocol. Protein extraction, SDS-PAGE, and western blot Proteins were extracted from 2 OD 600 units of yeast cells as described in ref. [54] . Protein extracts were loaded on precast Mini-PROTEAN TGX precast gels (Bio-Rad). Proteins were blotted on a nitrocellulose membrane with the Trans-Blot Turbo Transfer System (Bio-Rad). The membrane was fixed with Ponceau S solution (P7170, Sigma Aldrich) and blocked for 1 h with 5% skim milk in 1xPBS containing 0.001% Tween-20 (PBS-T). The primary antibodies were incubated overnight in 5% skim milk in PBS-T. Peroxidase coupled secondary antibodies were incubated for 1 h at room temperature. Antibodies are listed in Supplementary Data 4 . Antibodies were used in the following dilutions: anti-Rad53 (Abcam, Cat#ab166859, dilution 1:1000), Rabbit Peroxidase Anti-Peroxidase soluble complex (Sigma-Aldrich, Cat#P1291, dilution 1:2000), Mouse monoclonal anti-Phosphoglycerate Kinase 1 (22C5D8) (Invitrogen, Cat#459250, dilution 1:10,000), Mouse anti-Myc-Tag (9811) (Cell Signalling, Cat#2276S, dilution 1:1000), Goat Immun-Star anti-mouse (GAM)-HRP conjugate (Bio-Rad, Cat#170-5047, dilution 1:3000), Goat Immun-Star anti-rabbit (GAR)-HRP conjugate (Bio-Rad, Cat#170-5046, dilution 1:3000). The western blots were developed using the Super Signal West Pico Chemiluminescent Substrate (Thermo Scientific) and the ChemiDoc™ Touch Imaging System (Bio-Rad). Construction of strains with auxin-inducible degron Strains carrying the auxin-inducible degron (AID*) for RNase H2 (catalytic subunit Rnh201) were created as described before [27] . Plasmids and oligonucleotides are listed in Supplementary Data 3 . Construction of the cell cycle restricted RNase H2 alleles The S-RNH202-TAP-HIS3 and G2-RNH202-TAP-HIS3 alleles were described previously [8] . The G1-RNH202-TAP-HIS3 allele was created by amplifying the “G1 cassette” using the oligos oNA21 and oNA22 with the template pBL603 (containing the SIC1 promoter, the first 315 bp of the SIC1 gene and the NAT resistance cassette) [55] by PCR [56] . Transformed colonies were grown under selective pressure, and sequence verified by sequencing with the respective oligonucleotide pairs. The cell cycle specific expression was confirmed by western blot. Plasmids and oligonucleotides are listed in Supplementary Data 3 . α-factor arrest and release For cell cycle analysis, cells were synchronized in G1 phase by addition of 4 µg/mL α-factor (Zymo research, mating hormone peptide) for 2 h. Cells were then spun and washed three times with water, released into fresh YPD medium and further grown at 25 °C in a water bath. Protein and Flow cytometry samples were collected at indicated time points. Canavanine mutagenesis assay The CAN1 fluctuation analysis was performed as described in [57] . Relevant genotypes for the Can R mutation assay were streaked out 48 h prior inoculation to conserve population doublings within replicates. At least 14 independent single colonies from each genotype were entirely excised from the agar plate using a sterile scalpel to inoculate a 10 ml of YPD medium. The cultures were incubated at 30 °C, 250 rpm for 16 h. After measuring the optical density of the cultures they were harvested by centrifugation. Then, each culture was resuspended in 1 ml sterile water. Exactly 1 ml of each resuspension was transferred to a new tube. From this, a 10-fold dilution series up to a dilution factor of 10 6 was performed in a 96-well plate. Finally, 100 µl of all strains from the 10 −6 dilution were plated on a YPD plate and distributed with exactly four glass beads per plate. All strains were plated on SC-ARG plates supplemented with 60 µg/mL canavanine with the indicated dilution factor. The plates were incubated for 72 h at 30 °C before the outgrown colonies were manually counted. The medium for the Can R mutation assay was mixed, autoclaved and poured each day before plating to maintain constant conditions between replicates. For evaluation, the number (#) of mutant cells per culture, representing r , was calculated: 
    r=culturevol.×(conc. factor×#mutant colonies/plated vol.×dilution factor(plated))
 (1) The following correction was used to account for the progenies of each individual CAN1 mutation event per cell. With M being a scaled value that represents the number of cells that have actually undergone a mutation event (from which the counted progenies originated): 
    r=M(1.24+lnM)
 (2) The final mutation rate was calculated dividing M by the total number of cells present in the initial culture: 
    mutation rate=M/#cells in the culture
 (3) The data was plotted as the Median with 95% Confidence interval using the GraphPad PRISM8 software. Plating assay Exponential cultures at 30 °C were synchronized with α-factor for 1 h and then split to start the degradation of Rnh201-AID*-9Myc with 1 mM IAA (auxin) in 50% of the samples during the residual 1 h of synchronization. Half of the culture remained arrested in G1 phase and the other half was released into S phase, by washing out α-factor, in the presence or absence of 1 mM auxin for 30 min. Of each culture and condition, a suitable dilution was empirically determined that yielded in 100–200 colonies per YPD agar plate after outgrowth. The plates were incubated for 2 days at 30 °C. Colonies of 7 replicates were manually counted and adjusted for differences in optical density (OD 600 ) before dilution. Statistical analysis and plot generation was performed using Prism8 (GraphPad Software). Yeast spot assay Single colony derived yeast cells were incubated overnight at the appropriate temperature in liquid medium. Cells were diluted to 0.5 OD 600 and spotted in ten-fold serial dilutions onto YPD plates, SC plates, or plates containing the indicated amount of genotoxic drugs, i.e., methylmethanesulfonate (MMS), camptothecin (CPT) or hydroxyurea (HU) (all drugs: Sigma-Aldrich). The agar plates were incubated at the indicated temperatures and time and imaged using the ChemiDoc™ Touch Imaging System (Bio-Rad). Standard YPD agar has pH 5.5. To make YPD agar plates with alkaline pH, we titrated melted YPD agar with 10 N NaOH until pH 8.0 was reached. The wsc1::KAN knockout strain was used as a positive control for the alkaline agar plates [28] . Liquid yeast growth curves Yeast cells were diluted to 0.05 OD 600 in 100 µl of liquid growth medium, or medium containing drugs at indicated concentrations and transferred to a 96-well plate (Falcon®). Hourly OD 600 measurements were performed at 30 °C for 20 h by using a Tecan Spark® microplate reader. Growth curves were evaluated in Microsoft Excel. The linear range of each curve was plotted to find the linear fit with the formula y=Ye^Bx. The PD was determined using the log naturalis ln=0.6931 and the formula PD = ln/B*60 min. The PD plots were generated in GraphPad PRISM8. Alkaline gel electrophoresis Analysis of alkaline-labile sites in genomic DNA was performed as reported earlier [1] . Briefly, overnight cultures were diluted for exponential growth in 50 ml medium and harvested at the optical density of OD 600 = 0.6. Genomic DNA was isolated with the Qiagen Gentra Puregene Yeast/Bact Kit (Qiagen, 158567). The gDNA concentration was determined by an intercalating fluorescent dye supplied via the Qubit dsDNA broad-range kit (Invitrogen, Q32854). In a final volume of 40 µl, 10 µg of extracted gDNA were treated, shielded from light, for 2 h at 55 °C with 0.3 M KOH or 0.3 M KCl. KOH treated DNA samples were mixed with 8 µl 6× alkaline loading buffer (300 mM KOH, 6 mM EDTA, 18% (w/v) Ficoll Type 400, 0.15% (w/v) bromocresol green, 0.25% (w/v) xylene cyanol) before loading on a 1% alkaline agarose gel; the alkaline gel was casted using the 1× dilution of the 10× alkaline running buffer (0.5 mM NaOH, 10 mM EDTA). The alkaline gel was run in 1× alkaline running buffer. The KCl treated gDNA samples were loaded on a 1% TBE agarose gel with standard loading dye. Both gels were run at room temperature for 5 min at 65 V before reducing the voltage to 26 V for 18 h. The alkaline gel was neutralized in two washes of 250 ml (700 mM Tris-HCl pH 8.0, 1.5 M NaCl) for 45 min each with gentle shaking. Both gels were stained in a 1:10,000 SyBr Gold solution (ThermoFisher, S11494) (diluted in 1×TBE for the neutral gel; diluted in water for the alkaline gel) for 2 h with gentle shaking before image acquisition. Construction of cell cycle regulated RNH202 allele in the SGA query strain background The G1-RNH202-TAP (this study) , S- , and G2-RNH202-TAP alleles [8] were crossed to the haploid background strain (Y8205, Source C. Boone) for the SGA query strain construction. Selection of diploids, sporulation and tetrad analysis generated the four query strains used in SGA analysis. Cell cycle restricted protein expression of Rnh202 was confirmed by arrest and release experiment and western blot analysis. The selectable markers for SGA analysis were verified by PCR (oMT86/oMT91 for can1Δ::STE2pr-Sp_his5 , oMT89/oMT90 for lyp1Δ::STE3pr-LEU2 ) and replica-plating on YPD + (50 μg/ml canavanine, 50 μg/ml thialysine). The yeast strains are listed in Supplementary Data 2 . Synthetic genetic array (SGA) screen procedure and data evaluation The G1- , S- , and G2-RNH202-TAP query strains and a wild type RNH202 control query were crossed with the haploid genome-wide library of yeast gene deletion mutants, the YKO [58] . Crosses were performed in 1536-colony format, with the four queries combined on each screen plate, with four technical replicates of each cross, arranged next to each other. To minimize spatial effects, four outer rows and columns contained dummy strains. Mating, sporulation and selection of haploids carrying both a query allele (cell cycle regulated RNH202 alleles or wild type control) and a gene deletion were performed by sequential pinning of yeast colonies on appropriate selective media using a RoToR pinning robot (Singer Instruments) as described [59] . Plates with the final colony arrays were imaged after 24 h with the Singer PhenoBooth colony imager. Data analysis was performed in R (R Core Team (2021). R: A language and environment for statistical computing. http://www.R-project.org/ ) as detailed in https://github.com/Khmelinskii-Lab/nick_lesion_repair_SGA_screen . Briefly, photographs of colony arrays were segmented using the gitter package [60] to determine colony size. Measurements of empty positions and four outer rows and columns were assigned NA values. Colony size measurements on each plate were corrected for spatial effects using the SGA tools package [60] and normalized to the median on each plate. Genetic interactions in double mutants were identified under the assumption of multiplicative combination of effects of single mutants in the absence of genetic interactions [59] . For that, normalized colony size measurements were divided by the median per query to obtain normalized double mutant fitness. For each mutant in the YKO collection, differences between crosses with a cell cycle and the wild type queries were assessed with a t-test, excluding replicates contributing more than 90% of variance. The p -values were adjusted for multiple testing using the Benjamini-Hochberg method. Finally, replicates were summarized by their mean, excluding replicates contributing more than 90% of variance (Supplementary Data 5 ). Negative genetic interactions were verified through manual generation of haploid double mutants, by crossing single colonies from the YKO haploid collection to the S-RNH202 allele, selection for diploids, sporulation and tetrad analysis. False positives and linked genes have been excluded in the final analysis (greyed out). Materials Materials such as antibodies, enzymes, and chemicals are listed in Supplementary Data 4 . Reporting summary Further information on research design is available in the Nature Portfolio Reporting Summary linked to this article.